Coherent electron–phonon coupling in tailored quantum systems The coupling between a two-level system and its environment leads to decoherence. Within the context of coherent manipulation of electronic or quasiparticle states in nanostructures, it is crucial to understand the sources of decoherence. Here we study the effect of electron–phonon coupling in a graphene and an InAs nanowire double quantum dot (DQD). Our measurements reveal oscillations of the DQD current periodic in energy detuning between the two levels. These periodic peaks are more pronounced in the nanowire than in graphene, and disappear when the temperature is increased. We attribute the oscillations to an interference effect between two alternative inelastic decay paths involving acoustic phonons present in these materials. This interpretation predicts the oscillations to wash out when temperature is increased, as observed experimentally. Coherent spin manipulation has already been accomplished in AlGaAs/GaAs double quantum dots (DQDs) [1] , [2] and, more recently, also in InAs nanowires (NWs) [3] . Although the coherence times are usually limited by random nuclear fields [4] , also electron–phonon coupling can be a source of decoherence [5] . InAs NWs and graphene are two alternative and promising materials for achieving coherent spin manipulation. In InAs NW DQDs, spin-orbit interactions are very strong and enable a more efficient electron-spin resonance driven by spin-orbit interaction compared with AlGaAs/GaAs DQDs [3] . In graphene, it is expected that hyperfine coupling as a source of decoherence is very weak compared with AlGaAs/GaAs. Although electron–phonon interaction effects have been observed in carbon nanotube [6] , [7] , AlGaAs/GaAs [8] , or silicon quantum dots (QDs) [9] and in AlGaAs/GaAs DQDs [10] , [11] , only little is known about electron–phonon interaction in graphene and InAs NWs. Almost 60 years ago, Dicke [12] predicted superradiant and subradiant spontaneous emission, which was observed 40 years later with two trapped ions [13] . In this experiment, the spontaneous emission rate Γ( R ) of a two-ion crystal excited by a short laser pulse was studied as a function of the ion–ion separation R . Superradiant (subradiant) spontaneous emission was observed with Γ( R )>Γ 0 (Γ( R )<Γ 0 ), where Γ 0 is the emission rate of a single ion. In analogy to the Dicke subradiance phenomenon, Brandes et al . [14] later proposed an interference effect due to electron–phonon interactions in a solid-state two-level system (DQD). Our experimental observations are interpreted in this framework. Here, we report on an effect associated with coherent electron–phonon coupling in two entirely different DQD systems and therefore different electronic and phononic environments. The very strong confinement of electronic states in these two materials, in contrast to AlGaAs/GaAs DQDs, has enabled us to observe this coherent coupling, the solid-state analogue of the Dicke subradiance phenomenon. Our measurements show periodic oscillations in the current through both double dot systems as a function of the energy difference of the levels in the two dots. The energy dependence of these oscillations allows us to infer a coherent coupling between electrons and the phonon field. We find an enhancement of the coherent oscillations in the InAs NW compared with graphene in agreement with dimensional considerations. The temperature at which the experimentally detected oscillations disappear (≈600 mK) clearly supports the relevance of a coherent effect in the coupled electron–phonon system. Finally, this study shows new possibilities for using graphene and InAs NWs as nanoelectromechanical devices and, more specifically, as phonon detectors. 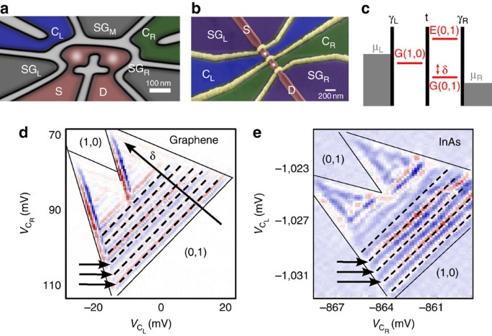Figure 1: Current in graphene and NW DQDs. (a) Schematic representation of the graphene DQD. The two dots are separated by a 30 nm wide constriction and connected to source and drain (in red) by 20 nm wide constrictions. Both constrictions, in blue and green, serve as side gates to control the electrochemical potential of the QDs as well as charge detectors for the QDs. Additional side gates are shaded in grey. (b) Tilted scanning electron microscopy image of the NW DQD. The InAs NW (in red) is deposited on an AlGaAs/GaAs heterostructure with a two-dimensional electron gas 37 nm below the surface. Again, the constrictions in blue and green serve as side gates and as charge detectors. The purple side gates offer additional tunability. Metallic top gates (in yellow) enable us to independently tune the tunnel barriers. (c) Energy-level diagram of the DQD at finite bias for non-zero detuning. (d) Graphene DQD: close-up of one pair of triple points forVbias=6 mV atT=120 mK (axisVCRis upside-down). The numerical derivative of the current with respect toVCRandVCLis plotted to highlight the periodic lines parallel to the base line. (e) InAs DQD: close-up of one pair of triple points forVbias=2.5 mV at 130 mK. The numerical derivative of the current with respect toVCRandVCLis plotted. Observation of periodic oscillations The two investigated devices are shown in Figure 1a (graphene) and Figure 1b (InAs NW). The current through a DQD is maximal at triple points of the charge stability diagram, in which the electrochemical potentials of both dots are degenerate and aligned with the electrochemical potentials of source and drain [15] . The schematic configuration of the DQD is illustrated by the energy-level diagram in Figure 1c . In Figure 1d,e , we show the numerical derivative of the current with respect to V CR and V CL , ∂ 2 I /∂ V CR ∂ V CL , for one pair of triple points in each material system. A bias voltage V bias =6 mV (graphene) and 2.5 mV (NW) has been applied across the DQDs, which results in a triangular shaped region of allowed transport. Figure 1: Current in graphene and NW DQDs. ( a ) Schematic representation of the graphene DQD. The two dots are separated by a 30 nm wide constriction and connected to source and drain (in red) by 20 nm wide constrictions. Both constrictions, in blue and green, serve as side gates to control the electrochemical potential of the QDs as well as charge detectors for the QDs. Additional side gates are shaded in grey. ( b ) Tilted scanning electron microscopy image of the NW DQD. The InAs NW (in red) is deposited on an AlGaAs/GaAs heterostructure with a two-dimensional electron gas 37 nm below the surface. Again, the constrictions in blue and green serve as side gates and as charge detectors. The purple side gates offer additional tunability. Metallic top gates (in yellow) enable us to independently tune the tunnel barriers. ( c ) Energy-level diagram of the DQD at finite bias for non-zero detuning. ( d ) Graphene DQD: close-up of one pair of triple points for V bias =6 mV at T =120 mK (axis V CR is upside-down). The numerical derivative of the current with respect to V CR and V CL is plotted to highlight the periodic lines parallel to the base line. ( e ) InAs DQD: close-up of one pair of triple points for V bias =2.5 mV at 130 mK. The numerical derivative of the current with respect to V CR and V CL is plotted. Full size image Along the baseline of the triangles (in Fig. 1d,e ), the two ground-state levels G(1,0) and G(0,1) are aligned and δ =0. We can roughly estimate the number of electrons in each InAs NW dot to N ~30. In graphene, a similar estimation is very difficult as we do not know exactly where the Dirac point is located. For a detuning δ ≠0, inelastic transitions are probed: if energy can be exchanged with the environment, a current flows as observed in Figure 1d,e . A striking feature is the presence of periodic peaks parallel to the baseline, indicated by arrows in Figure 1d,e , with a periodicity δ 0 =430 μeV (graphene, first cool down) and a smaller periodicity δ 0 =190 μeV (NW). These periodic current modulations have been observed in different triangles, in both bias directions with equal periodicity, and in two different cool downs (for graphene). For a more detailed analysis of similarities and differences between graphene and InAs NW DQDs, the currents through the DQDs along the detuning line (indicated in Fig. 1d ) have been measured ( Fig. 2 ) in a different triangle. As in the previous measurement, we observe that the periodicity in graphene is larger (270 μeV) than in the InAs NW (200 μeV). The periodic peaks are more pronounced in the InAs NW than in graphene. In total, we have measured four pairs of triple points for different gate configurations in graphene and have extracted δ 0 ≈430 μeV for the first cool down and δ 0 ≈220−280 μeV for the second cool down. In the InAs NW, we have measured 19 different triple points, 15 being in a range of δ 0 ≈150−215 μeV. These values are much smaller than the typical excited state energies, which are several meV above the ground state (see Fig. 2a,b ), because of the small effective mass m *≈0.02 m 0 (refs 16 , 17 ). In graphene, measurements realized in a single dot of similar size show excitations at energies of around 2–4 meV (refs 18 , 19 ). In the measured device, we see current steps superimposed on the periodic current oscillations at energies of 2 meV. We attribute the stepwise current increase to the opening of additional transport channels due to excited states, with comparable energies as measured in single dots. In the following, we provide evidence that our observations are related to an interference effect. 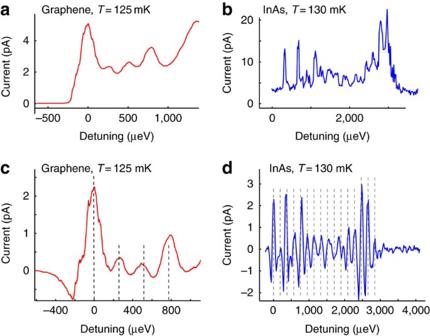Figure 2: Periodic oscillations in the current. (a) Raw experimental data: current through the graphene DQD along the detuning line for a bias voltageVbias=−5 mV atT=125 mK. (b) Raw experimental data: current through the InAs NW DQD along the detuning line for a bias voltageVbias=3 mV atT=130 mK. (c) Current through the graphene DQD along the detuning line (smoothed and background subtracted with an adjacent averaging algorithm). A periodicity of about 270 μeV can be observed. (d) Current through the InAs DQD along the detuning line (smoothed and background subtracted). We observe pronounced periodic oscillations with an amplitude of few pA. Figure 2: Periodic oscillations in the current. ( a ) Raw experimental data: current through the graphene DQD along the detuning line for a bias voltage V bias =−5 mV at T =125 mK. ( b ) Raw experimental data: current through the InAs NW DQD along the detuning line for a bias voltage V bias =3 mV at T =130 mK. ( c ) Current through the graphene DQD along the detuning line (smoothed and background subtracted with an adjacent averaging algorithm). A periodicity of about 270 μeV can be observed. ( d ) Current through the InAs DQD along the detuning line (smoothed and background subtracted). We observe pronounced periodic oscillations with an amplitude of few pA. Full size image Features of the coherent coupling To understand these observations, we model inelastic transitions, which occur in a DQD. We first suppose that for inelastic transitions phonons are emitted [11] . Therefore, the transition rates are proportional to the Bose–Einstein coefficient. For graphene, the coupling of acoustic phonons to electrons is due to deformation potential coupling [20] , [21] , [22] . The double dot is modelled as a two-level system with a bonding state |Ψ + = c L |L − c R | R and an antibonding state |Ψ − = c R |L − c L | R with | c L | 2 +| c R | 2 =1. We are interested in transitions between these two states due to the absorption or emission of acoustic phonons. The relevant matrix element for this process is Ψ + | e i qr |Ψ − , where e i qr arises from the Hamiltonian that describes the electron–phonon coupling. Emission and absorption rates due to the deformation potential coupling can be written as [23] where M is the single atom mass, N the number of atoms in the system and Δ the energy splitting between the two levels. To simplify | Ψ + | e iqr |Ψ − | 2 , we make two assumptions. First, we neglect the overlap between the electronic wave functions of the two dots, which is equivalent to saying that the cross terms ( c 2 R L | e iqr | R − c 2 L R | e iqr | L ) can be neglected compared with the direct terms c R c L ( L | e iqr | L − R | e iqr | R ). This gives Ψ + | e iqr |Ψ − = c R c L ( L | e iqr | L − R | e iqr | R ), that is, there are two alternative decay paths. In a second step, we assume that r | L = φ ( r ), where φ ( r ) describes a state localized in the left dot, which typically has an exponential decay at the dot boundaries, and r | R = φ ( r − d ) the state in the right dot, with d being the distance vector between the two dots. From this, we obtain the relation R | e iqr | R = e iqd L| e iqr | L . We finally have Ψ + | e iqr |Ψ − = c R c L L | e iqr | L (1− e iqd ), and therefore Γ abs/em | Ψ + | e iqr |Ψ − | 2 (1−cos( qd )). This expression predicts periodic oscillations in the emission rate as a function of quasi-momentum q , which can be interpreted as an interference effect in which the electron relaxes in either the left or right dot, analogous to the Dicke subradiant spontaneous decay [12] , [14] . The phase difference between the two interfering paths is related to the phonon wave function and the opposite parity of ground- and excited state (see Fig. 3a ). 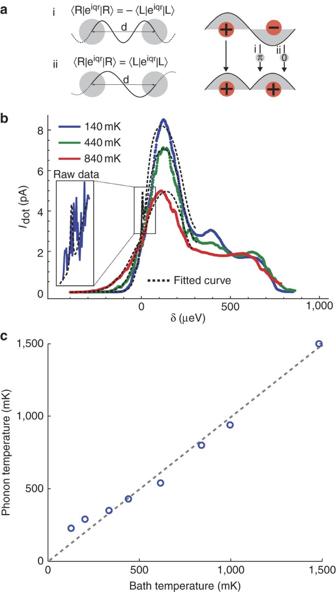Figure 3: Interaction with a bosonic environment. (a) Intuitive picture of the interference-based interpretation of the phonon effect. Depending on whether the distance between both dots is an even or an odd multiple of half a phonon wavelength, the phonon-mediated transition will shift the overall phase of the electronic wavefunction byk×2π (case ii) or (k+1/2)×2π (case i). In the antibonding state, transitions change the overall phase by π, in the bonding state the phase remains unchanged for an electron in the different spatial eigenstates. Overall, this leads to constructive interference in the right dot for case i (wavefunctions in phase) and destructive interference for case ii (phase difference of π). (b) Current through the graphene DQD as a function of the detuning between the two dots forVbias=−1 mV. Experimental data (solid lines): inelastic transitions close toδ=0 are strongly affected by temperature, as expected if we suppose a bosonic environment. The overall current is also modified as the coupling to the leads is slightly changed by temperature. Fitted curve (dashed lines): our model includes deformation potential coupling to phonons, coupling to the leads and the phonon absorption and emission rates. The broadening atδ=0 comes from the temperature dependence of the phonon absorption and emission rates, given by the Bose–Einstein distribution. Inset: the main figure shows averaged measurements (the measurements have been repeated five times), which wash out the elastic transition atδ=0. If we focus on a single measurement (as shown here), we observe a peak at zero detuning in most measured curves. (c) From the fitted curves we extract the phonon temperatures plotted as a function of bath temperature. Figure 3: Interaction with a bosonic environment. ( a ) Intuitive picture of the interference-based interpretation of the phonon effect. Depending on whether the distance between both dots is an even or an odd multiple of half a phonon wavelength, the phonon-mediated transition will shift the overall phase of the electronic wavefunction by k ×2π (case ii) or ( k +1/2)×2π (case i). In the antibonding state, transitions change the overall phase by π, in the bonding state the phase remains unchanged for an electron in the different spatial eigenstates. Overall, this leads to constructive interference in the right dot for case i (wavefunctions in phase) and destructive interference for case ii (phase difference of π). ( b ) Current through the graphene DQD as a function of the detuning between the two dots for V bias =−1 mV. Experimental data (solid lines): inelastic transitions close to δ =0 are strongly affected by temperature, as expected if we suppose a bosonic environment. The overall current is also modified as the coupling to the leads is slightly changed by temperature. Fitted curve (dashed lines): our model includes deformation potential coupling to phonons, coupling to the leads and the phonon absorption and emission rates. The broadening at δ =0 comes from the temperature dependence of the phonon absorption and emission rates, given by the Bose–Einstein distribution. Inset: the main figure shows averaged measurements (the measurements have been repeated five times), which wash out the elastic transition at δ =0. If we focus on a single measurement (as shown here), we observe a peak at zero detuning in most measured curves. ( c ) From the fitted curves we extract the phonon temperatures plotted as a function of bath temperature. Full size image The periodicities in graphene allow to extract a distance between the two dots of d =144 nm (first cool down) and d =220−280 nm (second cool down) for a sound velocity of v =15×10 3 m s −1 (25% below the theoretical predictions [21] ) and d =96−137 nm for a sound velocity v =5×10 3 m s −1 (ref. 16 ) in the InAs NW DQD. In both cases, our results are in agreement with the geometry of the DQDs (in the graphene DQD, we have measured a mutual coupling energy E m c ,1 ≈2.4 meV (first cool down) E m c ,2 ≈1.7 meV (second cool down) in agreement with a larger effective distance between the two dots for the second cool down). In a recent pioneering experiment realized in an InAs NW DQD with a diameter of 50 nm [16] , similar equidistant peaks with a separation δ ≈180−200 μeV were observed. The authors argue that these resonance lines result from a modified phononic energy spectrum due to the strong radial confinement. Following this argument, we should observe a separation δ ≈70−75 μeV in our measurements, considering that our NW is thicker (130 nm). Instead, we measure (at different triple points and for different gate configurations) δ ≈150−215 μeV. We also find that the periodicity δ is strongly affected by the electrostatic potential of our gates (not shown), although the phonon energy spectrum should not depend on the electronic environment. Thus, we conclude that the interpretation related to simple phonon confinement [16] cannot explain our measurements. Nevertheless, our interference-based approach could be in agreement with Weber et al . 's [16] observations of a separation of δ ≈180−200 μeV. Comparison between InAs NW and graphene The measurements of Figure 2c,d indicate that the interference effect is more pronounced in the InAs NW than in graphene. Different mechanisms could lead to such an observation. For instance, the assumption of localized electronic wavefunctions without overlap could be less relevant in graphene leading to a damping of the oscillations. In addition to this, the dimensionality of the system could influence the amplitude of the interference. In a two-dimensional system for example, the oscillatory part will be proportional to , where c λ is the sound velocity and θ is the angle between the quasi-momentum q and the distance vector d . In an ideal one-dimensional system we would obtain a factor , which implies more pronounced interference. Theoretical calculations which compare the phonon spectrum in a graphene and in an InAs NW DQD are needed to further clarify this point. Signatures of a bosonic environment In the solid-state environment of our DQDs, temperature is expected to antagonize interference effects by destroying coherence. In the phonon absorption and emission rates (Eq. 1), temperature only appears through the Bose–Einstein distribution with Γ em ( n +1), Γ abs n , and n =1/( e Δ/ kT −1) where is the energy difference between the bonding and antibonding state, t the tunnel coupling between the dots, and δ = E L − E R the energy difference between left and right states [24] . Measurements of the current through the graphene DQD close to δ ~0 μeV for different temperatures are shown in Figure 3b . We observe a clear dependence of the inelastic transitions on temperature, and as expected the current for negative detuning is enhanced at elevated temperatures as absorption is more pronounced when the temperature is increased. For more quantitative predictions, we calculate the expected current through the DQD: the rate equations for the occupation of the states can be expressed as a function of the tunnel coupling, Γ L (left barrier), Γ R (right barrier), Γ em (emission) and Γ abs (absorption), allowing to calculate the stationary solution [25] . The stationary current is plotted as a function of detuning δ in Figure 3b (dashed line) for a bath temperature of ~140 mK. The good agreement with the measured curve enables us to extract a phonon temperature of ~230 mK. The discrepancy between bath and phonon temperatures disappears when the mixing chamber temperature is increased, as can be seen in Figure 3c , where the extracted phonon temperatures are plotted as a function of bath temperature. Above 300 mK, bath and phonon temperatures are in excellent agreement. This result confirms an energy-exchange with the phonon bath. 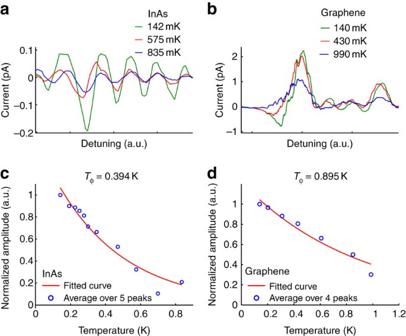Figure 4: Temperature dependence of current oscillations. (a) InAs DQD: current oscillations with background subtracted using an adjacent averaging algorithm, for different temperatures as a function of detuning. A magnetic field of 1 T is applied to have a better resolution of the peaks. (b) Graphene DQD: current oscillations with background subtracted, for different temperatures as a function of detuning. (c) Normalized amplitude of the oscillations as a function of temperature for the InAs DQD (quasi-1D system). The blue circles represent the normalized oscillation amplitude, averaged over the first five maxima. The red solid line is a exp(−T/Tφ)-fit, yieldingTφ=394 mK. (d) Normalized amplitude of the oscillations, averaged over the first four maxima, as a function of temperature for the graphene DQD (two-dimensional system). The average temperature dependence of the first four peaks is similar and can be fitted with an exp(−T/Tφ) (red solid line) behaviour withTφ=895 mK. Temperature dependence In Figure 4a and b , we plot the current oscillations for InAs and graphene DQDs, respectively, for temperatures from 140 mK up to 1 K. We note a continuous decrease of the peak amplitudes with increasing temperature. These observations confirm the difference compared with the interpretation in ref. 16 : current replica due to the interaction between electrons and individual phonon modes should not depend strongly on temperature below 1 K ( δ 0 ≈200 μeV≈2.3 K). Figure 4: Temperature dependence of current oscillations. ( a ) InAs DQD: current oscillations with background subtracted using an adjacent averaging algorithm, for different temperatures as a function of detuning. A magnetic field of 1 T is applied to have a better resolution of the peaks. ( b ) Graphene DQD: current oscillations with background subtracted, for different temperatures as a function of detuning. ( c ) Normalized amplitude of the oscillations as a function of temperature for the InAs DQD (quasi-1D system). The blue circles represent the normalized oscillation amplitude, averaged over the first five maxima. The red solid line is a exp(− T / T φ )-fit, yielding T φ =394 mK. ( d ) Normalized amplitude of the oscillations, averaged over the first four maxima, as a function of temperature for the graphene DQD (two-dimensional system). The average temperature dependence of the first four peaks is similar and can be fitted with an exp(− T / T φ ) (red solid line) behaviour with T φ =895 mK. Full size image The extracted temperature dependence of the average amplitude for the first five peaks (normalized by the lowest temperature amplitude) is presented in Figure 4c . The red solid line is a exp(− T / T φ )-fit to our data with T φ =394 mK as discussed below. A similar dependence is observed in graphene ( Fig. 4d ) with T φ =895 mK. To explain this temperature dependence, we consider decoherence: we suppose that the phase difference between the two interfering emission processes is not perfectly defined due to coupling to the thermal bath. In the limit, in which the thermal energy is large compared with the energy equivalent of the transition time scales ( in our case), phase fluctuations are given by the fluctuation-dissipation theorem and the visibility v of the oscillations decays exponentially over a characteristic temperature (ref. 26 ). The quantity T φ quantifies the strength of the thermal fluctuations the electron is experiencing in the interferometer (see Fig. 3a ). As decoherence of the phonon wave function is quite unlikely, we think that with increasing temperature bonding and antibonding states are washed out. However, theoretical calculations are needed to validate this hypothesis. In conclusion, we have observed an oscillatory effect in transport through DQDs in graphene and in an InAs NW, which we attribute to coherent electron–phonon coupling in nanostructured geometries. The characteristic phase difference for this interference is determined by the phonon field phase difference between both dots. We have observed that the effect is more pronounced in an InAs NW compared with a graphene DQD. Finally, we have shown that the temperature dependence of these oscillations is compatible with a thermal decoherence mechanism. This study may contribute to a better understanding of the role of the phonon bath in electron transport through NWs and graphene DQDs. Fabrication . The procedures to fabricate our graphene quantum system are described in refs 27 , 28 . The InAs NW, grown by metal organic vapor-phase epitaxy, is deposited on a predefined Hall bar of an AlGaAs/GaAs heterostructure with a two-dimensional electron gas (2DEG) 37 nm below the surface. The etching mask for the DQD and detector structure, realized by electron beam lithography, is designed in such a way that the trenches in the 2DEG forming the detectors and the constrictions in the NW are aligned (see Fig. 1b ) [29] . Applying a voltage between each detector and the corresponding QD enables us to control the electrochemical potentials of the QDs [30] . To tune the tunnel barriers independently, the trenches in the 2DEG are additionally filled with metallic top gates (AlOx/Al/Ti/Au). The two dots have a lithographic dimension of roughly 100 nm for the graphene DQD and 130 nm for the InAs NW. The measurements were performed in two different dilution refrigerators at 120 mK (base temperature). How to cite this article: Roulleau, P. et al . Coherent electron–phonon coupling in tailored quantum systems. Nat. Commun. 2:239 doi: 10.1038/ncomms1241 (2011).